Self-assembled hydrogels utilizing polymer–nanoparticle interactions Mouldable hydrogels that flow on applied stress and rapidly self-heal are increasingly utilized as they afford minimally invasive delivery and conformal application. Here we report a new paradigm for the fabrication of self-assembled hydrogels with shear-thinning and self-healing properties employing rationally engineered polymer–nanoparticle (NP) interactions. Biopolymer derivatives are linked together by selective adsorption to NPs. The transient and reversible interactions between biopolymers and NPs enable flow under applied shear stress, followed by rapid self-healing when the stress is relaxed. We develop a physical description of polymer–NP gel formation that is utilized to design biocompatible gels for drug delivery. Owing to the hierarchical structure of the gel, both hydrophilic and hydrophobic drugs can be entrapped and delivered with differential release profiles, both in vitro and in vivo . The work introduces a facile and generalizable class of mouldable hydrogels amenable to a range of biomedical and industrial applications. Hydrogels comprise an important class of material well-suited for a range of applications on account of their high water content and highly tunable mechanical properties [1] , [2] , [3] , [4] . Many hydrogel systems utilize covalent crosslinking approaches [5] , including radical processes initiated by light [6] , [7] , temperature [8] and pH [9] . These covalently crosslinked hydrogels form robust, tough and elastic materials; however, they can be limited by the irreversibility of their crosslinks. Mouldable hydrogels that can be formed and processed prior to use and subsequently applied in a conformal manner provide attractive alternatives to covalent hydrogels for many applications, including local drug delivery in the body, cell carriers for tissue engineering, bone fillers or hydraulic fracturing fluids. To serve these functions, mouldable hydrogels must exhibit viscous flow under shear stress (shear-thinning) and rapid recovery when the applied stress is relaxed (self-healing). In addition, it is extremely beneficial if the high shear viscosity is low for facile application through high gauge needles. These properties enable minimally invasive implantation in vivo though direct injection or catheter-based delivery, contributing to a rapid gain in interest in their use for controlled drug delivery [10] . Self-assembly via non-covalent crosslinking provides a route to fabricate mouldable and injectable hydrogels with shear-thinning and self-healing properties arising from strong, yet transient and reversible crosslinks [2] , [10] . Several systems have been reported utilizing natural host–guest or receptor–ligand pairs, such as (strep)avidin with biotin [11] , [12] , leucine zipper [13] , [14] and ‘dock-and-lock’ [15] , [16] protein structures prepared with genetic engineering techniques, or with synthetic macrocyclic host molecules, such as cyclodextrins [17] , [18] or cucurbit[ n ]urils [19] , [20] , [21] , [22] , [23] . In each of these examples, self-assembly of functional materials via non-covalent, intermolecular interactions with dynamic and reversible macroscopic behaviour was exploited. However, the shear-thinning and self-healing hydrogels presented to date are limited by poor mechanics and slow self-healing or require challenging, costly and poorly scalable synthesis of macromolecular components through protein engineering or complex, multi-step chemical functionalization. Crucial requirements to the biomedical translation of mouldable and injectable hydrogels are facile and mild formation, modular modification and finely tunable control over mechanical properties, as well as rapid self-healing following injection. Within the field of self-assembly, polymer–nanoparticle (NP) interactions have arisen as a simple route to assemble tunable and self-healing polymeric materials without the need for complex synthetic approaches or specialized small-molecule binding partners [24] , [25] . For example, complementary affinity between polymers (molecular binders) and the surface of hard NPs (clay nanosheets/silicates) has been utilized to fabricate high-water-content and mouldable hydrogels [24] , [26] , [27] , [28] . More recently, NP adsorption to polymer gels has been exploited to achieve strong, rapid adhesion between disparate gels [25] . A similar phenomenon has been exploited to enhance the bulk mechanical properties of polysaccharide-based, physically crosslinked hydrogels by incorporating drug-loaded poly(lactic- co -glycolic acid) microspheres into the hydrogel formulation [29] , [30] . Inspired by these elegant approaches, we synthesize shear-thinning and self-healing hydrogels in a mild, modular and scalable manner based solely on interactions between cellulose derivatives and NPs for biomedical applications. Herein, we report the preparation and application of hydrogels driven by non-covalent interactions between hydroxypropylmethylcellulose derivatives (HPMC- x ) and core-shell NPs ( Fig. 1 ; Supplementary Fig. 1 ). Transient and reversible interactions between the NPs and HPMC chains govern polymer–NP (PNP) hydrogel self-assembly, allowing for flow under applied stress and complete recovery of their structural properties when the stress is relaxed. PNP hydrogels are formulated with poly(ethylene glycol)- block -poly(lactic acid) (PEG- b -PLA) NPs to enable dual loading of a hydrophobic molecule into the PEG- b -PLA NPs and a second, hydrophilic molecule into the aqueous bulk of the gel. PEG- b -PLA PNP hydrogels are biocompatible and afford differential release of multiple compounds in vivo following subcutaneous implantation. 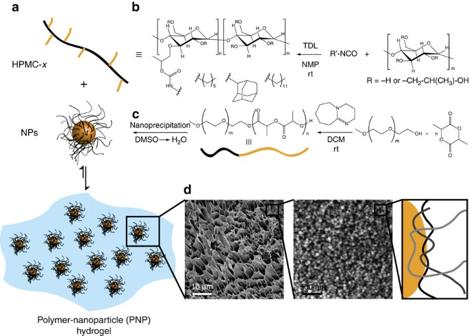Figure 1: Fabrication of PNP hydrogels from HPMC derivatives and nanoparticles. (a) Schematic representation of the preparation of polymer–nanoparticle (PNP) hydrogels utilizing non-covalent interactions between core-shell nanoparticles (NPs) and (b) hydrophobically modified hydroxypropylmethylcellulose. (c) The NPs can be composed of either poly(styrene) (PS; non-degradable) or poly(ethylene glycol)-block-poly(lactic acid) (PEG-b-PLA; biodegradable). (d) Cryogenic scanning electron microscopy images of PNP gels composed of PSNPs (d~50 nm) demonstrate a homogeneous distribution of NPs within the gel structure, indicating that the network is held together by multivalent, dynamic polymer–nanoparticle interactions (as illustrated; polymer chains, grey scale; nanoparticle, orange). Figure 1: Fabrication of PNP hydrogels from HPMC derivatives and nanoparticles. ( a ) Schematic representation of the preparation of polymer–nanoparticle (PNP) hydrogels utilizing non-covalent interactions between core-shell nanoparticles (NPs) and ( b ) hydrophobically modified hydroxypropylmethylcellulose. ( c ) The NPs can be composed of either poly(styrene) (PS; non-degradable) or poly(ethylene glycol)- block -poly(lactic acid) (PEG- b -PLA; biodegradable). ( d ) Cryogenic scanning electron microscopy images of PNP gels composed of PSNPs ( d ~50 nm) demonstrate a homogeneous distribution of NPs within the gel structure, indicating that the network is held together by multivalent, dynamic polymer–nanoparticle interactions (as illustrated; polymer chains, grey scale; nanoparticle, orange). Full size image PNP hydrogels Initially, PNP hydrogels were formed by mixing aqueous solutions of HPMC ( M n ~700 kDa) and commercially available carboxy-functionalized polystyrene NPs (PSNPs; D H ~50 nm; 1 wt% HPMC: 10 wt% PSNPs) under ambient conditions ( Fig. 2a ). These gels formed rapidly on mixing and exhibited a shear storage modulus of G ′=140 Pa. For these studies, storage modulus ( G ′) was used as a measure of hydrogel strength, and tan δ, which is the ratio of the loss modulus ( G ″) over the storage modulus (tan δ = G ″/ G ′), was used as a measure of hydrogel elasticity. HPMC was chosen as the primary polymer for preparation of PNP hydrogels on account of its high solubility, molecular weight, functionality and biocompatibility [31] . PSNPs enabled a systematic investigation of the effect of NP number and NP diameter ( D H ~50 to 500 nm), with uniform surface properties, on PNP gel formation. Hydrogel formation is exclusive to the presence of both PSNPs and HPMC as PSNPs (10 wt%) and HPMC (1 wt%) solutions alone are each low viscosity liquids. Cryogenic transmission electron microscopy (TEM) indicates that the NPs remain homogeneously dispersed in the gel state, suggesting that gel formation is driven by PNP interactions and not agglomeration ( Supplementary Fig. 8 ). Moreover, HPMC combined with commercially available silica NPs (Ludox TM-50; d ~22 nm; 1 wt% HPMC: 10 wt% NPs) failed to form a gel. These data indicated that selective adsorption of HPMC chains to PSNPs results in crosslinking and gel formation. 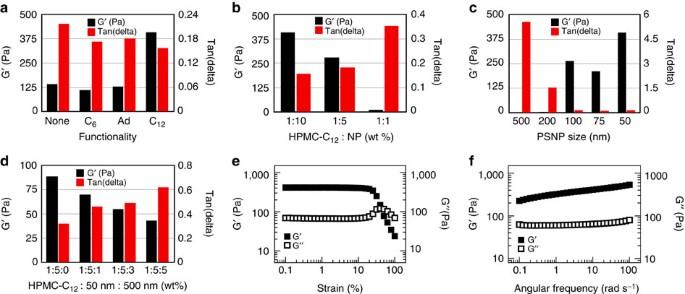Figure 2: Rheological characterization of PNP hydrogels from HPMC derivatives and nanoparticles. Oscillatory rheological properties of hydrogels from (a) HPMC-xbearing various functionality (0.5 mmol g−1; 1 wt%) with PSNPs (50 nm; 10 wt%), (b) HPMC-C12with PSNP (50 nm) at various loadings and (c) HPMC-C12(1 wt%) with PSNPs (10 wt%) of various sizes. All values collected atω=10 rad s−1,, 25 °C. (d) Oscillatory rheological properties of hydrogels from HPMC-C12(1 wt%) with PSNPs of two different sizes: 50 nm (5 wt%) and 500 nm (1, 3 and 5 wt%). The large particles () contribute to a dramatic decrease in the mechanical properties of the PNP gels, even though more particles are being added to the formulation and thus contributing to an increase in the number of polymer–nanoparticle interactions per unit volume (n). (e) Strain-dependent (ω=10 rad s−1, 25 °C) and (f) frequency-dependent (, 25 °C) oscillatory shear rheology of HPMC-C12(1 wt%)/PSNP (10 wt%) hydrogels. Figure 2: Rheological characterization of PNP hydrogels from HPMC derivatives and nanoparticles. Oscillatory rheological properties of hydrogels from ( a ) HPMC- x bearing various functionality (0.5 mmol g −1 ; 1 wt%) with PSNPs (50 nm; 10 wt%), ( b ) HPMC-C 12 with PSNP (50 nm) at various loadings and ( c ) HPMC-C 12 (1 wt%) with PSNPs (10 wt%) of various sizes. All values collected at ω =10 rad s −1 , , 25 °C. ( d ) Oscillatory rheological properties of hydrogels from HPMC-C 12 (1 wt%) with PSNPs of two different sizes: 50 nm (5 wt%) and 500 nm (1, 3 and 5 wt%). The large particles ( ) contribute to a dramatic decrease in the mechanical properties of the PNP gels, even though more particles are being added to the formulation and thus contributing to an increase in the number of polymer–nanoparticle interactions per unit volume ( n ). ( e ) Strain-dependent ( ω =10 rad s −1 , 25 °C) and ( f ) frequency-dependent ( , 25 °C) oscillatory shear rheology of HPMC-C 12 (1 wt%)/PSNP (10 wt%) hydrogels. Full size image Efficient crosslinking necessitates strong affinity between the NPs and the polymer chains, that is, the free energy gain ( ε ) resulting from adsorption of a polymer chain to the surface of a NP should be greater than or comparable to the thermal energy ( k B T ). In addition, the average number of interactions per polymer chain and particle must be >2 to achieve percolation of the network. Moreover, to favour polymer bridging of multiple NPs (as opposed to polymer wrapping around individual particles), the NP diameter should be comparable to, or less than, the persistence length ( l P ) of the polymer strands. When these criteria are met, NPs are able to serve as crosslinkers between the polymer chains, while the polymer chains may bridge many different particles, enabling hydrogel formation. From polymer physics, the modulus ( G ) of PNP hydrogels can be related to the number of PNP interactions per unit volume ( n ) and the energy associated with each interaction ( αk B T ) using theoretical tools analogous to those developed for covalent hydrogels: G ≈ n · αk B T (ref. 32 ). Based on this physical picture of PNP hydrogels, we hypothesized that hydrophobic modification of HPMC (yielding HPMC- x ) could be exploited to increase the energy associated with each PNP interaction ( αk B T ), thereby increasing the modulus of the gel given the same number of interactions per unit volume. In this manner, modification would facilitate favourable interactions between the hydrophobic moiety on the HPMC chain and the hydrophobic core of the PSNPs, thereby enhancing the adsorption energy of the HPMC to the NPs. HPMC was readily functionalized using commercially available isocyanates (including hexyl, adamantyl and dodecyl isocyanate; Supplementary Table 1 ) in a one-step reaction performed at ambient temperature using dibutyltin dilaurate (TDL) as a catalyst [33] . PNP gels were then formulated with HPMC- x , where x refers to hexyl (C 6 ), adamantyl (Ad) or dodecyl (C 12 ) functionality, and PSNPs ( D H ~50 nm; 1 wt% HPMC- x : 10 wt% PSNPs). PNP gels formed with either HPMC-C 6 or HPMC-Ad possessed similar properties to unmodified HPMC gels. However, PNP gels formed with HPMC-C 12 were roughly three times stronger ( G ′=400 Pa), indicating an increased interaction energy between the C 12 moieties and the PSNPs ( Fig. 2a ; Supplementary Fig. 2 ). These observations are particularly appealing as the rheology of the HPMC-C 12 polymer at 1 wt% is characteristic of a low viscosity fluid, despite conjugation of hydrophobic moieties ( Supplementary Fig. 3 ) and the polymer’s ability to form hydrogels at higher concentrations [34] . In addition, we investigated the effect of NP number and size on PNP gel formation. We hypothesized that gel modulus would scale directly with the number of NPs and that particle sizes below a critical diameter, expected to be comparable to the persistence length of the polymer ( l P ~90 nm for HPMC) to facilitate bridging between particles, would favour gel formation. The number of NPs in the PNP gels was modulated by formulating PNP solutions with decreasing fractions of PSNPs (1 wt% HPMC-C 12 : 10, 5 or 1 wt% PSNPs with D H ~50 nm). The shear storage modulus ( G ′) decreased, as predicted, with fewer NPs, and consequently decreasing number of PNP interactions per unit volume ( n ; Fig. 2b ). Next, we screened PNP gel formation with PSNPs of various sizes ( D H ~50, 75, 100, 200 and 500 nm; 1 wt% HPMC-C 12 : 10 wt% PSNPs). We observed that robust gels formed with particle diameters ≤100 nm, whereas larger particles failed to produce gels ( Fig. 2c ). These observations support our hypothesis that D H ≤ l P favour gel formation; yet, this set of experiments was confounded by the fact that as particle diameter increases for a given loading, the particle number decreases ( Supplementary Fig. 4 ). To elucidate further the effect of particle size on PNP gel formation, we formulated a PNP gel composed of HPMC-C 12 (1 wt%) and both 50 nm PSNPs (5 wt%) and 500 nm PSNPs (1, 3 and 5 wt%). As large particles were titrated into the PNP gels, a monotonic decrease in material properties was observed ( Fig. 2d ), highlighting the importance of the critical particle size in PNP gel formulations. Strain-dependent oscillatory rheology ( Fig. 2e ) of the HPMC-C 12 PNP gels (1 wt% HPMC-C 12 : 10 wt% 50 nm PSNPs) displayed an extremely broad linear viscoelastic region in addition to network failure at high strains, indicating a wide processing regime and shear-thinning behaviour. The frequency dependence of the storage and loss oscillatory shear moduli ( G ′ and G ″, respectively) confirmed hydrogel-like behaviour as G ′ is dominant across the whole range of frequencies observed (0.1–100 rad s −1 ; Fig. 2f ). Step-strain measurements were then performed to investigate the recovery of material properties following network rupture at high strains (a critical parameter for injectability). A high magnitude strain ( ) was applied to break the hydrogel structure, followed by a low magnitude strain ( ) to monitor the rate and extent of recovery of bulk properties ( Fig. 3a ). These materials exhibited exceptionally fast and complete recovery of properties within seconds following stress-induced flow. Moreover, the rate and extent of recovery was unchanged over several cycles of breaking and reforming, highlighting the reversible and robust nature of the non-covalently crosslinked hydrogel structure ( Fig. 3b ). 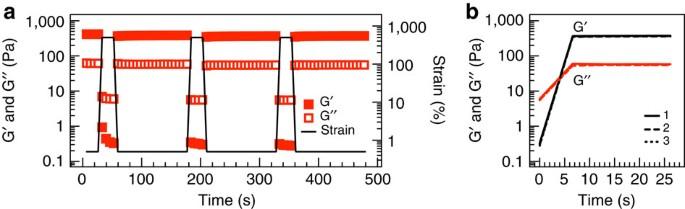Figure 3: Shear-thinning and self-healing behaviour of PNP hydrogels. (a) Step-strain measurements of HPMC-C12(1 wt%)/PSNP (10 wt%) hydrogels over three cycles (ω=10 rad s−1, 25 °C) with (b) overlayed zoom of the recovery of material properties after each cycle. Figure 3: Shear-thinning and self-healing behaviour of PNP hydrogels. ( a ) Step-strain measurements of HPMC-C 12 (1 wt%)/PSNP (10 wt%) hydrogels over three cycles ( ω =10 rad s −1 , 25 °C) with ( b ) overlayed zoom of the recovery of material properties after each cycle. Full size image The rheology of PNP gels supports the physical picture of gel assembly. Polymer adsorption to core-shell NPs drives PNP formation. Gel properties are influenced by the energetic favourability of adsorption (enhanced by hydrophobicity of the HPMC), number of PNP interactions, as well as the diameter of the NPs. Moreover, the transient and reversible nature of polymer adsorption to the NPs imparts the PNP gels with shear-thinning and rapid self-healing properties. When the hydrogel is strained, chains adsorbed to the particles are under tension and detach from the particle surface to relax this tension. In this manner, polymer–NP interactions retard failure and ensure strong crosslinking as the energy dissipated during the stress-induced desorption is much greater than ε ~ k B T . In addition, these interactions allow the gel to flow with sufficient applied stress (shear-thinning) as polymers desorb and slide past one another. On relaxation of the applied stress, the gel rapidly re-forms (self-healing) as polymers adsorb to particles in a new configuration. PNP hydrogels from biodegradable NPs With robust design principles in hand, we sought to develop PNP gels composed of biocompatible and biodegradable NPs. PEG- b -PLA core-shell NPs have been employed as drug delivery vehicles in a range of in vivo applications [35] , [36] and presented as a promising candidate for PNP gels as they can be formed with D H ~100 nm in a reproducible and scalable manner. PEG 5k - b -PLA 20k block copolymers were prepared via organocatalytic ring opening polymerization utilizing 1,8-diazabicyloundec-7-ene (DBU) as a catalyst ( Fig. 1c ) [37] . Core-shell NPs ( D H ≈100 nm according to dynamic light scattering (DLS)) were prepared by nanoprecipitation of the amphiphilic diblock copolymer from dimethyl sulfoxide (DMSO; a good solvent for both blocks) into water (a selective solvent for the hydrophilic PEG block) [38] . These synthetic protocols are facile, rapid and are easily scaled. As with PSNPs, mixing aqueous solutions of HPMC-C 12 and PEG- b -PLA NPs produced a PNP hydrogel (HPMC-C 12 1 wt%: PEG- b -PLA NPs 10 wt%) with analogous mechanical properties ( Fig. 4a,b ). The presence of the PEG corona on the NPs dramatically reduced the inherent affinity between the HPMC and the NPs, resulting in a 30-fold increase in shear storage modulus with conjugation of C 12 moieties relative to non-functionalized HPMC ( Fig. 4a ). Thus, strong adhesion between HPMC- x polymers and PEG- b -PLA NPs, and consequent hydrogel formation, requires the presence of a sufficiently long hydrophobic tail. Moreover, decreasing the size of the PEG corona on the NPs by employing block copolymers with a shorter PEG chain (PEG 2k - b -PLA 16k ) led to enhanced PNP interactions and stronger materials ( Supplementary Fig. 6 ). Furthermore, the dynamic nature of the non-covalent interactions was retained in these materials, affording similar stress-induced flow properties and material recovery as for hydrogels formulated with PSNPs ( Fig. 4c,d ). The shear-thinning behaviour on these materials was further investigated with steady shear measurements ( Supplementary Fig. 7 ), which indicated a large change in the viscosity (Δ η ~10 3 Pa s) from low to high shear rates, a beneficial property for facile injection through high gauge needles. 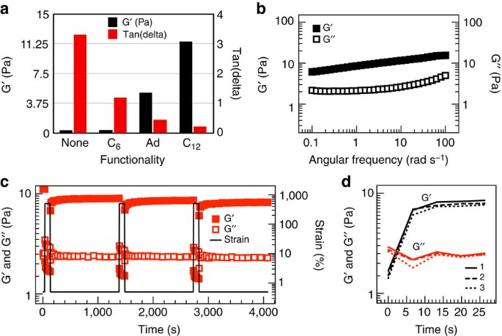Figure 4: Rheological characterization of biodegradable PNP hydrogels. (a) Oscillatory rheological properties (ω=10 rad s−1,, 37 °C) of hydrogels from HPMC-xbearing various functionality (0.5 mmol g−1; 1 wt%) with PEG-b-PLA NPs (10 wt%;). (b) Frequency-dependent (, 37 °C) oscillatory shear rheology of HPMC-C12(1 wt%)/PEG-b-PLA NPs (10 wt%) hydrogels. (c) Step-strain measurements of HPMC-C12(1 wt%)/PEG-b-PLA NPs (10 wt%) hydrogels over three cycles (ω=10 rad s−1, 37 °C) with (d) overlayed zoom of the recovery of material properties after each cycle. Figure 4: Rheological characterization of biodegradable PNP hydrogels. ( a ) Oscillatory rheological properties ( ω =10 rad s −1 , , 37 °C) of hydrogels from HPMC- x bearing various functionality (0.5 mmol g −1 ; 1 wt%) with PEG- b -PLA NPs (10 wt%;). ( b ) Frequency-dependent ( , 37 °C) oscillatory shear rheology of HPMC-C 12 (1 wt%)/PEG- b -PLA NPs (10 wt%) hydrogels. ( c ) Step-strain measurements of HPMC-C 12 (1 wt%)/PEG- b -PLA NPs (10 wt%) hydrogels over three cycles ( ω =10 rad s −1 , 37 °C) with ( d ) overlayed zoom of the recovery of material properties after each cycle. Full size image In vitro controlled drug release As PNP hydrogels composed of PEG- b -PLA NPs contained both hydrophilic and hydrophobic domains, we hypothesized that dual encapsulation and controlled release of therapeutics was possible with these materials ( Fig. 5a ). Moreover, as the PEG- b -PLA NPs constituted a structural component of the gel, we sought to characterize the gel’s ability to impart differential release characteristics to multiple cargo. We first encapsulated fluorescein isothiocyanate-labelled bovine serum albumin (BSA–FITC), a model protein therapeutic, into the aqueous phase of the hydrogels by dissolving it into the HPMC-C 12 solution prior to hydrogel formation. The BSA was completely retained within the hydrogels on formation, and the release of the BSA into water was monitored using ultraviolet–visible (UV-Vis) spectroscopy. The release profile ( Fig. 5b ) appeared to be first order and governed by Fickian diffusion [39] . Modelling of the release data according to the Ritger–Peppas equation [40] confirmed diffusional release ( k =0.031±0.001% per h; Fig. 5c ). 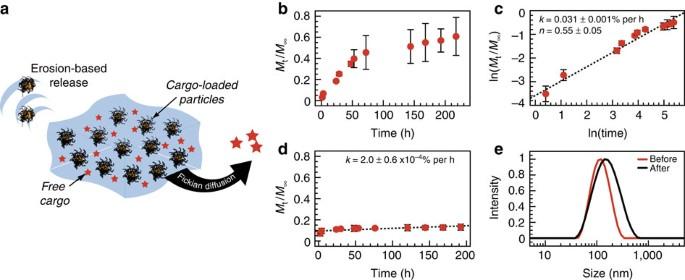Figure 5:In vitrocontrolled delivery by differential mechanisms simultaneously. (a) Schematic representation of two stage release of therapeutic cargo. (b) Drug release profiles of Bovine Serum Albumin (BSA; hydrophilic) from hydrogels showing the cumulative proportion of ‘drug’ released (Mt/M∞; the cumulative fractional mass released at timet;n=3; data presented as mean±s.e.m.). (c) Fitting of the release data indicated that BSA was released from the hydrogel by Fickian diffusion with a diffusional release coefficient,k, of 0.031±0.001% per h. (d) Drug release profile of Oil Red (OR; hydrophobic) from hydrogels prepared with OR-loaded PEG-b-PLA NPs (n=3; data presented as mean±s.e.m.). In this case, OR was released exclusively by erosion from the hydrogel surface (k=2.0±0.6 × 10−4% per h) following a small burst release (<10%). (e) Dynamic light scattering (DLS) characterization of PEG-b-PLA NPs (as prepared before hydrogel formation) and the supernatant following erosion of PNP hydrogels (that is, after release of NPs) supported the proposed erosion-based release mechanism. Figure 5: In vitro controlled delivery by differential mechanisms simultaneously. ( a ) Schematic representation of two stage release of therapeutic cargo. ( b ) Drug release profiles of Bovine Serum Albumin (BSA; hydrophilic) from hydrogels showing the cumulative proportion of ‘drug’ released ( M t / M ∞ ; the cumulative fractional mass released at time t ; n =3; data presented as mean±s.e.m.). ( c ) Fitting of the release data indicated that BSA was released from the hydrogel by Fickian diffusion with a diffusional release coefficient, k , of 0.031±0.001% per h. ( d ) Drug release profile of Oil Red (OR; hydrophobic) from hydrogels prepared with OR-loaded PEG- b -PLA NPs ( n =3; data presented as mean±s.e.m.). In this case, OR was released exclusively by erosion from the hydrogel surface ( k =2.0±0.6 × 10 −4 % per h) following a small burst release (<10%). ( e ) Dynamic light scattering (DLS) characterization of PEG- b -PLA NPs (as prepared before hydrogel formation) and the supernatant following erosion of PNP hydrogels (that is, after release of NPs) supported the proposed erosion-based release mechanism. Full size image In stark contrast to these observations, a model hydrophobic drug compound, Oil Red (OR), which was encapsulated into the PEG- b -PLA NPs during the nanoprecipitation process [38] prior to hydrogel formation, was released from the hydrogels with an entirely different profile ( Fig. 5d ). This model drug demonstrated a small burst release (<10%), followed by zero-order release ( k =2.0±0.6 × 10 −4 % per h), attributed to erosion-based release. Indeed, when the release supernatant was observed by DLS, NPs of a similar D H were observed, indicating that intact particles release from the gel through an erosion-based mechanism ( Fig. 5e ). Thus, PNPs exploit PEG- b -PLA NPs as a structural component of the material as well as a carrier motif allowing for multiple therapeutics to be encapsulated simultaneously and released with differential profiles. Previous studies with similar nanocomposite drug delivery systems, employing drug-loaded poly(lactic- co -glycolic acid) nanospheres as mechanical enhancers of physical hydrogel blends, have demonstrated release of both hydrophilic (1 to 4 days) and hydrophobic (up to 30 days) species in vitro [30] . In vivo implantation and controlled drug release Having synthesized injectable hydrogels with unique drug delivery profiles, we sought to characterize the in vivo utility of PNP gels (1 wt% HPMC-C 12 : 10 wt% PEG- b -PLA NPs). First, adult C57BL/6 mice were injected subcutaneously with PNP hydrogels and a phosphate-buffered saline (PBS) bolus as a control. While the PBS bolus dissipated in less than an hour, the PNP hydrogel, which reformed immediately following injection, remained intact at 7 days ( Supplementary Fig. 9 ). The injected materials were harvested after 3 and 7 days and histological anaylsis ( Fig. 6 ) demonstrated mild infiltration of the material by neutrophils at day 3, which were replaced primarily by macrophages at day 7. The material was beginning to clear by macrophages at this time, with no evidence of multi-nucleated giant cells or lymphocytes, no indication of fibrosis and no signs of inflammation or damage in the adjacent tissue (additional histological analysis is contained in Supplementary Figs 10 and 11 ). 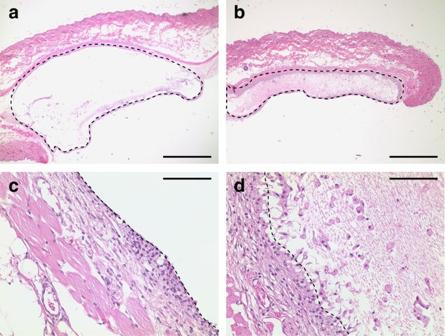Figure 6:In vivobiocompatibility. Histological anaylsis of haematoxylin stained samples taken after 3 days (a: × 2 andc: × 40) and 7 days (b: × 2 andd: × 40)in vivo. In each image, the interface between biological tissue and PNP gel is denoted with a dotted line. Scale bar, 2,000 μm (× 2) and 100 μm (× 40). Figure 6: In vivo biocompatibility. Histological anaylsis of haematoxylin stained samples taken after 3 days ( a : × 2 and c : × 40) and 7 days ( b : × 2 and d : × 40) in vivo . In each image, the interface between biological tissue and PNP gel is denoted with a dotted line. Scale bar, 2,000 μm (× 2) and 100 μm (× 40). Full size image Based on the favourable biocompatibilty of the gels, PNP gels were formulated with a model hydrophobic therapeutic (Texas Red conjugated to 1,2-dihexadecanoyl-glycero-3-phosphoethanolamine; TR) loaded into PEG- b -PLA NPs and a model hydrophilic protein therapeutic (Alexa Fluor 680 conjugated to BSA; BSA-AF) loaded into the aqueous bulk of the gel, to investigate their in vivo release characteristics. Adult SKH1E (hairless) mice were injected subcutaneously with these dual-‘therapeutic’-loaded PNP gels and the release was monitored via intravital fluorescence imaging ( Fig. 7a ). It was not possible to quantitatively investigate the release rate of the model therapeutics from the hydrogel in vivo on account of photobleaching of the TR dye and changing PNP hydrogel size on account of its mouldability. Yet, a consistent release pattern was observed in the SKH1E mice ( n =5) wherein the BSA accessed more of the animal than the TR. With a cut-off value of 20% relative intensity, fluorescent analysis revealed that the BSA was present ~10 mm from the injection site, whereas the TR remained within ~4 mm of the injection site ( Fig. 7b–d ). Control experiments with BSA-AF alone (bolus injection) and BSA-AF with HPMC-C 12 ( Supplementary Fig. 13 ) indicated that BSA release was governed primarily by interactions between BSA and HPMC-C 12 and not hydrogel network constraints. Furthermore, control experiments with TR-loaded particles alone ( Supplementary Fig. 14 ) highlight that PNP hydrogels enabled simultaneous release of both hydrophobic and hydrophilic molecular cargo in vivo from a single gel. 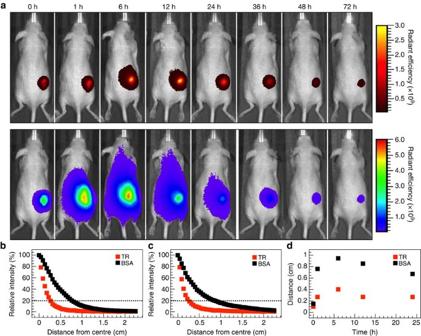Figure 7:In vivodual-therapeutic release. (a) Intravital fluorescence imaging of the release of TR-loaded NPs (top) and BSA-AF (bottom) from a single material. Plots of relative intensity of model therapeutic fluorescence versus distance from the centre of the hydrogel implant (n=5) at (b) 1 h and (c) 12 h. (d) Radius of release at 20% relative fluorescence intensity over time (n=5). Figure 7: In vivo dual-therapeutic release. ( a ) Intravital fluorescence imaging of the release of TR-loaded NPs (top) and BSA-AF (bottom) from a single material. Plots of relative intensity of model therapeutic fluorescence versus distance from the centre of the hydrogel implant ( n =5) at ( b ) 1 h and ( c ) 12 h. ( d ) Radius of release at 20% relative fluorescence intensity over time ( n =5). Full size image In summary, we prepare shear-thinning injectable hydrogels utilizing polymer–NP interactions between hydrophobically modified cellulose derivatives (HPMC- x ) and NPs. Transient and reversible hydrophobic forces between the NPs and HPMC chains govern the self-assembly of hydrogels, enabling them to flow under applied shear stress and facilitating complete recovery of their material properties in a matter of seconds when the stress is relaxed. Moreover, biocompatible hydrogels formulated with PEG- b -PLA NPs enable dual loading of a hydrophobic molecule into the PEG- b -PLA NPs and a second hydrophilic molecule into the aqueous bulk of the gel. Owing to the hierarchical structure of the gel, molecular delivery is controlled both by Fickian diffusion and erosion-based release affording differential release of multiple compounds from a single material, in vitro and in vivo . The biocompatibility of these materials and the differential release of multiple loaded model therapeutics is demonstrated in vivo . Overall, this manuscript demonstrates a class of injectable hydrogels for controlled drug delivery applications with facile synthesis and minimally invasive implantation in vivo . Instrumentation and materials 1 H NMR (400 MHz) spectra were recorded using a Bruker Avance QNP 400. Chemical shifts are recorded in p.p.m. ( δ ) in H 2 O with the internal reference set to δ =4.80 p.p.m. Attenuated total reflectance Fourier transform infrared (ATR FT-IR) spectroscopy was performed using a Perkin-Elmer Spectrum 100 series FT-IR spectrometer equipped with a universal ATR sampling accessory. Gel permeation chromatography (GPC) was carried out in either tetrahydrofuran (THF) on divinylbenzene columns or in H 2 O on glucose-modified divinylbenzene columns, both utilizing a Malvern Viscotek TDA 305 triple detection system. Samples were filtered over 0.2 μm polytetrafluoroethylene (when using THF) or polyvinylidenedifluoride (when using H 2 O) filters before injection using a 1.0 ml min −1 flow rate. Molecular weights and polydispersities were determined by comparing with either polymethylmethacrylate (when using THF) or dextran (when using H 2 O) standards. DLS measurements were performed with a Malvern Instruments Zetasizer Nano-ZS. Rheological characterization was performed using a TA Instruments AR-G2 stress controlled rheometer fitted with a Peltier stage. Dynamic oscillatory strain amplitude sweep measurements were conducted at a frequency of 10 rad s −1 (unless otherwise noted). Dynamic oscillatory frequency sweep measurements were conducted at a 2% strain amplitude (unless otherwise noted). All measurements were performed using a 20 mm, 4° cone geometry and analyzed using TA Instruments TRIOS software. Cryogenic scanning electron microscopy (CryoSEM) images of PNP gels where acquired using a Zeiss NVision 40 (Carl Zeiss SMT, Inc.) field emission scanning electron microscope at an acceleration voltage of 2 kV. To prepare samples for imaging ~100 μl of gel was transferred to a sample stub and then plunged into a slushy (liquid and solid) nitrogen bath. The samples where next transferred to an EM VCT100 vacuum cryo-transfer system (Leica Microsystems, Inc.) to selectively remove surface water (vitreous ice) by controlled specimen sublimation. The frozen sample were then further fractured with a sharp blade and sputter coated with a thin layer of platinum and palladium metals prior to imaging. Cryogenic TEM (CryoTEM) images where acquired using a JEOL 2100 FEG microscope (Jeol Inc. Peabody, MA, USA) equipped with an Gatan 2kx2k UltraScan CCD camera at an acceleration of 200 kV and at magnification ranges of × 10,000– × 30,000. To prepare samples for imaging, ~3 μl of NP suspensions was transferred to a lacey copper grid (coated with continuous carbon). Next, using a Gatan Cryo Plunge III the grids where blotted with great care to remove any excess liquid without causing damage to the carbon layer. The prepared grids where then mounted on a Gatan 626 cryo-holder equipped in the TEM column. The specimen and holder tips were next cooled down using liquid nitrogen, and subsequently transferred to the CryoTEM for imaging. Monomethoxy-PEG (5 kDa) was purchased from Aldrich and was purified by azeotropic distillation with toluene. Lactide (LA) was purchased from Aldrich and dried in a desiccator over P 2 O 5 prior to use. Carboxy-functional PSNPs were purchased from Phosphorex and used as received. All other materials were purchased from Aldrich and used as received. General synthesis of HPMC- x polymers HPMC (1.0 g) was dissolved in N -methylpyrrolidone (NMP; 45 ml) by stirring at 80 °C for 1 h. Once the solution had cooled to room temperature, a solution of 1-hexylisocyanate, 1-adamantylisocyanate or 1-dodecylisocyanate (0.5 mmol) and triethylamine (2 drops) were dissolved in N -methylpyrrolidone (5 ml) and added to the reaction mixture, which was then stirred at room temperature for 16 h. This solution was then precipitated from acetone and the polymer was recovered by filtration, dried under vacuum at room temperature for 24 h and weighed, yielding the functionalized HPMC as a white amorphous powder (0.96 g, 96%). FT-IR: . PEG- b -PLA synthesis PEG (0.25 g, 4.1 mmol) and DBU (10.6 mg, 10 μl, 1.0 mol% relative to LA) were dissolved in dichloromethane (DCM; 1.0 ml). LA (1.0 g, 6.9 mmol) was dissolved in DCM (3.0 ml) with mild heating. The LA solution was then added rapidly to the PEG/DBU solution and was allowed to stir rapidly for 10 min. The reaction mixture was then quenched by addition of acetone (7.0 ml) and the PEG- b -PLA copolymer was recovered by precipitation from cold diethyl ether, collected by filtration and dried under vacuum to yield a white amorphous polymer (1.15 g, 92%). GPC (THF): M n (PDI)=25 kDa (1.09). PEG- b -PLA NP preparation A solution of PEG-PLA in DMSO (40 mg ml −1 ) was added dropwise to water (10 × v/v) under a high stir rate. NPs were purified by ultracentrifugation over a filter (molecular weight cut-off of 10 kDa; Millipore Amicon Ultra-15) followed by resuspension in water to a final concentration of 150 mg ml −1 . NP size and dispersity were characterized by DLS. PNP gel preparation PNP gels were prepared by first dissolving HPMC polymers in water (30 mg ml −1 ) with stirring and mild heating. NPs were either purchased or prepared according to literature procedures [38] and were concentrated to 15 wt% solutions. HPMC polymer solution (150 μl) and NP solution (300 μl) were then added together and mixed well by vortex (some samples were mildly centrifuged to remove bubbles arising from mixing). In vitro release Two experiments were designed to investigate encapsulation and release of a hydrophobic molecule (OR) and a hydrophilic molecule (BSA-FITC). For the first experiment, hydrogels were prepared as mentioned above except with BSA-FITC dissolved alongside the HPMC polymer, resulting in a final concentration of BSA-FITC of 1 wt% in the hydrogel. For the second experiment, OR-loaded PEG-PLA NPs were prepared by co-nanoprecipitation of OR with PEG-PLA block copolymer. These NPs were then used to prepare hydrogels as above. Hydrogel of either type (200 μl) was placed into a 1.5 ml centrifuge tube and deionized water (1.3 ml) was added on top of the hydrogel. This set-up was placed into an incubator at 37 °C and 1 ml of the aqueous supernatant solution was replaced with fresh deionized water at predetermined time intervals. The collected aqueous solutions were analyzed for solute concentration based on calibration curves prepared using either OR or BSA-FITC absorbance. All experiments were performed in triplicate. In vivo biocompatibility studies All animal procedures were performed according to MIT Animal Care and Use Committee approved protocols. For biocompatibility studies, adult male C57BL/6 mice (8 weeks old) were injected subcutaneously on the back with PNP gels (200 μl; HPMC-C 12 1 wt%: PEG- b -PLA NPs 10 wt%) using a 26G syringe. At 3 and 7 days following administration, mice were killed and the hydrogel and surrounding tissue were harvested (3 mice per time point). Tissue was fixed for 24 h in formalin and cross-sections of the skin and underlying material (~40 μm in thickness), embedded in paraffin, were stained with standard haematoxylin and eosin or Mason’s trichrome. In vivo release studies PNP gels were prepared with BSA-AF (10 μM in the final gel; Life Technologies) loaded into the aqueous phase and TR encapsulated within the PEG- b -PLA NPs ([TR]=10 μM in the final gel). Control hydrogels, containing only one of the fluorescent compounds, were similarly prepared. Adult male SKH1E mice (8 weeks old) were injected subcutaneously on the back with PNP gels (200 μl; HPMC-C 12 1 wt%: PEG- b -PLA NPs 10 wt%) using a 26G syringe. For in vivo imaging, 8-week-old male hairless SKH1E mice were first maintained on an alfalfa-free diet for 2 weeks prior to administration to limit background fluorescence. Mice were anesthetized using inhaled isoflurane, and 200 μl was injected subcutaneously into the rear right flank of the animal using a 26G syringe. Treatment groups consisted of the hydrogel with the combined fluorophores ( n =5), the control hydrogel with TR only ( n =2), the control hydrogel with BSA-AF only ( n =2), a bolus injection of TR-loaded NPs ( n =3), an injection of BSA-AF with HPMC-C 12 ( n =3) and a bolus injection of BSA-AF in PBS ( n =1). Imaging was conducted on an IVIS Spectrum in vivo imaging system with a heated stage and an inhaled isoflurane manifold. Fluorescent images were collected at several time points over the following week, using filter sets of 570/620 (TR) and 675/720 (AF-680) with a 1.5-cm subject height using small binning and an F-stop of 1. How to cite this article: Appel, E. A. et al . Self-assembled hydrogels utilizing polymer–nanoparticle interactions. Nat. Commun. 6:6295 doi: 10.1038/ncomms7295 (2015).